Impact of macromolecular crowding on DNA replication Enzymatic activities in vivo occur in a crowded environment composed of many macromolecules. This environment influences DNA replication by increasing the concentration of the constituents, desolvation, decreasing the degrees of freedom for diffusion and hopping of proteins onto DNA, and enhancing binding equilibria and catalysis. However, the effect of macromolecular crowding on protein structure is poorly understood. Here we examine macromolecular crowding using the replication system of bacteriophage T7 and we show that it affects several aspects of DNA replication; the activity of DNA helicase increases and the sensitivity of DNA polymerase to salt is reduced. We also demonstrate, using small-angle X-ray scattering analysis, that the complex between DNA helicase and DNA polymerase/trx is far more compact in a crowded environment. The highest enzymatic activity corresponds to the most compact structure. Better knowledge of the effect of crowding on structure and activity will enhance mechanistic insight beyond information obtained from NMR and X-ray structures. Enzymatic processes observed in dilute buffer are often assumed to represent those in the cellular environment. However, most often this is not the case as the cell is filled with macromolecules in high density, leading to macromolecular crowding [1] . The in vivo concentration of molecules in the cytoplasm is between 50 and 400 mg ml −1 , ~70% being proteins [2] . Such crowding affects enzymatic activities both in vitro and in vivo . It is not always feasible to study the macromolecules under cellular conditions. To mimic cellular conditions’ inert crowding agents such as polyethylene glycol, dextran and Ficoll are often used. Proteins can also be used as crowding agents with bovine serum albumin representing a common additive. There are many examples of the effect of co-solutes on the properties of macromolecules and protein–nucleic acid complexes [3] . These co-solutes are thought to mimic the crowding effect in the cell that arises from DNA, RNA and protein complexes. Macromolecular crowding and the thermodynamic effects have been recognized since the 1960s by the studies of Ogston [4] . Notwithstanding the wealth of information on the effect of macromolecular crowding, the effect of macromolecular crowding on structure–function relationships is poorly understood. Macromolecular crowding stabilizes the native state of a protein by destabilizing the unfolded state, thus compensating for the energetically unfavourable ‘folded’ conformation [5] , [6] . An experimental and computational analysis has examined the effect of macromolecular crowding on structural changes between the folded and unfolded states of apoflavodoxin. These studies demonstrated that the effects of macromolecular crowding on protein structure are observable [7] . To assess the interactions between DNA molecules Parsegian et al . applied osmotic pressure in ordered arrays of DNA molecules and used X-ray diffraction to measure the structural changes [8] . The osmotic pressure method they developed utilizes the equivalent of the mechanical work (osmotic pressure) needed to bring macromolecules closer in spite of their repulsive interactions and the chemical work (removing of the solute) needed to concentrate the macromolecular subphase. In a different instance using far-UV circular dichroism spectroscopy, Stagg et al . [9] showed the structural effects of elevated amounts of Ficoll 70 on apoflavodoxin. The theoretical radius of gyration ( R g ) of apoflavodoxin indicates compactness in the crowded environment. There are limited reports on the effect of molecular crowding on DNA replication. Previous studies revealed effects on several aspects of DNA metabolism among them: oriC replication [10] , blunt-end DNA ligation by DNA ligase [11] , activities of phage T4 DNA kinase [12] , the association of accessory proteins [13] and the assembly of a phage T4 DNA polymerase holoenzyme [14] . Macromolecular crowding has also been used as a tool to detect interactions within the T4 replisome [15] . In the present study, we examine the effect of macromolecular crowding on the proteins that mediate leading-strand DNA synthesis. Phage T7 has evolved an economical mechanism for the replication of its DNA [16] . In contrast to eukaryotes or even E. coli , where tens of proteins are required, in the T7 system only four proteins account for the major reactions that occur at the replication fork: (i) the gene 5 DNA polymerase (gp5), and (ii) its processivity factor, the host encoded thioredoxin (trx), (iii) the gene 4 helicase-primase (gp4) and (iv) the gene 2.5 ssDNA binding protein (gp2.5). The limited number of proteins enables: (1) reconstitution of a replisome, (2) determination of the structures of functional complexes, (3) examination of the composition of active replisomes and (4) studying the effect of macromolecular crowding. The structure of interacting species within the replisome is not known although extensive effort has been made in this direction [17] . Therefore, alternative methods that provide low resolution structure such as small-angle X-ray scattering (SAXS) are useful. Macromolecular crowding reduces diffusion A computer simulation of the random walk of lysozyme within the volume of an E. coli cell in the presence or the absence of 18,000 ribosomes is shown in Fig. 1a . Restriction of spatial movement caused by decreased diffusion is observed in the crowded environment. One important consequence of this effect is the stabilization of weakly bound complexes. In addition to the effect on diffusion, macromolecules occupy between 5 and 40% of the cell volume. This volume is not accessible to other molecules, and the resulting effect is designated as the excluded volume effect [18] , whose magnitude depends on the size of the molecule in question. Another major effect of macromolecular crowding is solvent entropy. In a mixture of macromolecules and smaller molecular components the loss of entropy of the large molecules is compensated by the gain in entropy of the smaller molecules. Thus, desolvation around macromolecules enhances the entropy that compensates for the loss in the conformational entropy that accompanies folding or complex formation (for review see Levy and Onuchic [19] ). 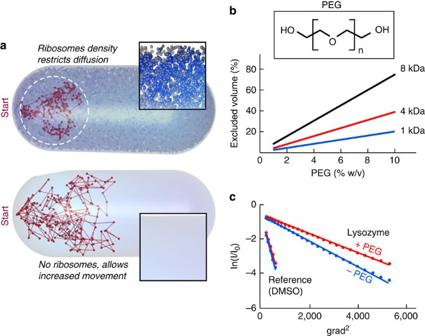Figure 1: Effects of macromolecular crowding. (a) Random walk in a crowded environment. Simulation for random walk (red) of a 30 kDa protein in the presence (upper panel) or absence (bottom panel) of 18,000 ribosomes as crowding agents in a volume of anE. colicell. The simulation was based on the calculation of diffusion coefficient using theD=(kBT)/3 πηd wherekBTis scaling factor of Boltzmann constant and the temperature,ηis a viscosity value for the interior of anE. colicell=3.5 × 10−3Kg m−1s−1(ref.48),dis the diameter of the particle used in the simulation=30 Å. The average displacement was computed as follows:A=2*R*D*τ, whereτis the interval for displacement=0.0001, s andRis the dimensions=3. (b) Calculation of the volume that PEG of different sizes (1, 4 and 8 kDa) occupies at different concentrations. At 4% (40 mg ml−1), PEG 1 kDa occupies 8% of the volume in a test tube; 4% PEG 1 kDa provides the approximate crowding effect foundin vivo(ref.47). (c) Translational diffusion of 1 mM lysozyme in the presence or the absence of 4% PEG 1 kDa determined using DOSY-NMR. The logarithm of the relative intensity is plotted against the square of the gradient strength ranging from 15 to 80 G cm−1. The decrease in magnetization with increasing gradient strength was analysed using the equation:whereDis the diffusion coefficient withkBis the Boltzmann constant,Tthe temperature,ηthe viscosity,Fthe dimensionless Perrin factor,rSthe hydrodynamic radius of the moleculeq=γδg, Δ=150 ms (separation of the gradient echo),δ=2.5 ms (gradient duration),γthe gyromagnetic ratio of the nucleus andgthe strength of the gradient (ranging from 15 to 80 G cm−1. Thirty two points were recorded in the indirect dimension. DMSO was used as an internal reference. Figure 1: Effects of macromolecular crowding. ( a ) Random walk in a crowded environment. Simulation for random walk (red) of a 30 kDa protein in the presence (upper panel) or absence (bottom panel) of 18,000 ribosomes as crowding agents in a volume of an E. coli cell. The simulation was based on the calculation of diffusion coefficient using the D =( k B T )/3 πηd where k B T is scaling factor of Boltzmann constant and the temperature, η is a viscosity value for the interior of an E. coli cell=3.5 × 10 −3 Kg m −1 s −1 (ref. 48 ), d is the diameter of the particle used in the simulation=30 Å. The average displacement was computed as follows: A =2* R * D * τ , where τ is the interval for displacement=0.0001, s and R is the dimensions=3. ( b ) Calculation of the volume that PEG of different sizes (1, 4 and 8 kDa) occupies at different concentrations. At 4% (40 mg ml −1 ), PEG 1 kDa occupies 8% of the volume in a test tube; 4% PEG 1 kDa provides the approximate crowding effect found in vivo (ref. 47 ). ( c ) Translational diffusion of 1 mM lysozyme in the presence or the absence of 4% PEG 1 kDa determined using DOSY-NMR. The logarithm of the relative intensity is plotted against the square of the gradient strength ranging from 15 to 80 G cm −1 . The decrease in magnetization with increasing gradient strength was analysed using the equation: where D is the diffusion coefficient with k B is the Boltzmann constant, T the temperature, η the viscosity, F the dimensionless Perrin factor, r S the hydrodynamic radius of the molecule q=γδg , Δ=150 ms (separation of the gradient echo), δ =2.5 ms (gradient duration), γ the gyromagnetic ratio of the nucleus and g the strength of the gradient (ranging from 15 to 80 G cm −1 . Thirty two points were recorded in the indirect dimension. DMSO was used as an internal reference. Full size image The most widely used crowding agent is polyethylene glycol (PEG). PEG is a straight-chain polymer containing simple repeating subunits; PEG 1 kDa, used in the present study, has 21 repeating units and is best modelled as a spherical particle [20] . PEG and other crowding agents can increase the rate of enzymatic reactions [21] , alter reaction products [1] , protect macromolecules from thermal denaturation [22] , accelerate protein folding [23] and facilitate nucleic acids renaturation [24] . PEG also induces precipitation of proteins at high concentration (30%) and is used in protein purification. We calculated the volume that PEG molecules of different sizes occupy at different concentrations ( Fig. 1b ). For example, at a concentration of 4% PEG 1 kDa, 8% of the solution is occupied by PEG. Macromolecular crowding alters the binding properties and rate constants of a number of enzymes including DNA polymerases. We have examined the effect of increasing the concentration of PEG on the structure of the replication proteins and on the reactions they catalyse. To determine if the macromolecular crowding effect of PEG is comparable to that found in vivo on the diffusion of a protein, we used NMR to measure the diffusion of lysozyme (15 kDa) ( Fig. 1c ). The diffusion coefficient in the presence of PEG is reduced 13-fold, a ratio similar to that observed in cells [25] . Macromolecular crowding enhances the activity of the gp5/trx complex The processivity factor, E. coli trx, binds with high affinity (5 nM) to T7 gp5 in a 1:1 stoichiometry [26] to increase the binding of gp5 to a primer-template 20–80-fold [26] . The increased affinity enhances the processivity of gp5 from <50 nucleotides (nt) per binding event to ~800 [26] resulting in a dramatic increase in the macroscopic rate of DNA synthesis. We have examined the effect of PEG on the polymerase activity of gp5 when mixed with trx in a ratio of 1:1 ( Fig. 2b , left). PEG increases the activity of gp5 as much as trx in the same molar ratio relative to gp5 ( Fig. 2b , right). 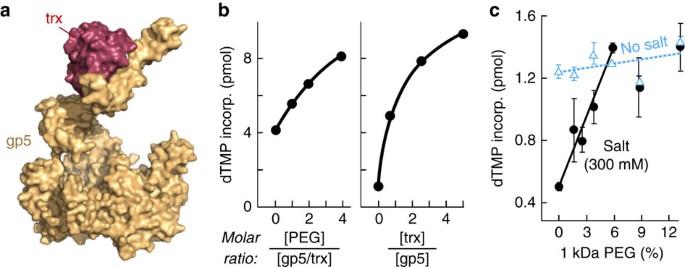Figure 2: Gp5/trx polymerase activity and macromolecular crowding. (a) T7 DNA polymerase (gp5, yellow) bound to its processivity factorE. colithioredoxin (trx, red) polymerizes nucleotides continuously on the leading strand. The crystal structure of gp5/trx bound to primer template and an incoming nucleotide (PDB id code: 1t8e (ref.34) in a view from the side. The figure was created using PyMOL (http://www.pymol.org). (b) Polymerase activity of gp5 with increasing amounts of trx (right). The activity was measured in a standard reaction containing 40 mM Tris-HCl (pH 7.5), 10 mM MgCl2, 10 mM DTT, 50 mM potassium glutamate, 0.25 mM dATP, dCTP, dGTP, and [α–32P] dTTP, 20 nM primed M13 DNA, 20 nM gp5 and the indicated amount of trx. After incubation at 37 °C for 10 min the amount of [α–32P] dTMP incorporated into DNA was measured. Increased polymerase activity of gp5 and trx premixed in a ration of 1:1 is observed as the content of PEG is increased (left). (c) Effect of macromolecular crowding by PEG on polymerase activity of gp5/trx in the presence or the absence of salt. Polymerase activity was measured under similar buffer conditions as ina. Gp5 (5 nM) was mixed with trx (25 nM) in the presence of 300 mM NaCl (black) or in absence of NaCl (cyan). The error bars were derived from three independent experiments. Figure 2: Gp5/trx polymerase activity and macromolecular crowding. ( a ) T7 DNA polymerase (gp5, yellow) bound to its processivity factor E. coli thioredoxin (trx, red) polymerizes nucleotides continuously on the leading strand. The crystal structure of gp5/trx bound to primer template and an incoming nucleotide (PDB id code: 1t8e (ref. 34 ) in a view from the side. The figure was created using PyMOL ( http://www.pymol.org ). ( b ) Polymerase activity of gp5 with increasing amounts of trx (right). The activity was measured in a standard reaction containing 40 mM Tris-HCl (pH 7.5), 10 mM MgCl 2 , 10 mM DTT, 50 mM potassium glutamate, 0.25 mM dATP, dCTP, dGTP, and [α– 32 P] dTTP, 20 nM primed M13 DNA, 20 nM gp5 and the indicated amount of trx. After incubation at 37 °C for 10 min the amount of [α– 32 P] dTMP incorporated into DNA was measured. Increased polymerase activity of gp5 and trx premixed in a ration of 1:1 is observed as the content of PEG is increased (left). ( c ) Effect of macromolecular crowding by PEG on polymerase activity of gp5/trx in the presence or the absence of salt. Polymerase activity was measured under similar buffer conditions as in a . Gp5 (5 nM) was mixed with trx (25 nM) in the presence of 300 mM NaCl (black) or in absence of NaCl (cyan). The error bars were derived from three independent experiments. Full size image We have shown previously that the activity of gp5/trx is reduced as the NaCl concentration is increased from 50 to 300 mM [27] . At 125 mM NaCl, gp5/trx retains 50% activity. The high salt presumably masks the charged residues at the DNA-binding surface. We proposed that the difference in the behaviour of gp5 and gp5/trx at high salt concentration arises from a different distribution of charged amino acids on the DNA-binding interface. The binding of trx to gp5 leads to a conformational change leading to a different electrostatic potential [27] . We examined the effect of PEG on the activity of gp5/trx in the absence or presence of 300 mM NaCl, a concentration that diminished the activity and the binding of gp5/trx to DNA in the earlier studies. Macromolecular crowding does not affect the processivity of DNA polymerase [15] and indeed increasing PEG concentrations result in only a slight (<10%) increase in polymerase activity in the absence of NaCl ( Fig. 2c , cyan). However, in the presence of 300 mM NaCl there is a three-fold increase upon the addition of PEG 1 kDa up to 4% where gp5/trx retains full activity ( Fig. 2c , black). Macromolecular crowding enhances helicase but not primase activity of gp4 Gp4 is a multifunctional enzyme bearing helicase and primase activities in the same polypeptide. We have used individual domains of gp4 to focus on specific activities ( Fig. 3a , bottom). Gp4A (residues 1–566, 63 kDa) is the full-length protein. Gp4B (residues 64–566, 56 kDa) arises from an internal initiation codon and is present in phage-infected cells in amounts equivalent to the full-length protein. Gp4B lacks the N-terminal zinc-binding subdomain, an essential component for primer synthesis. 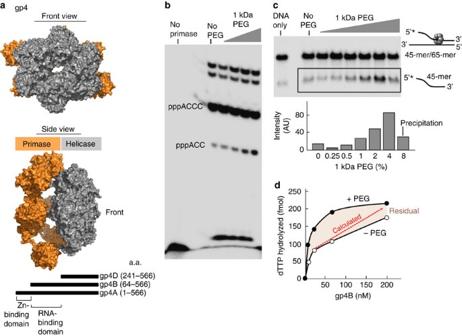Figure 3: The effect of macromolecular crowding on gp4 activity. (a) Front (top panel) and side view (middle panel)of a gp4 model. Gp4 has both primase and helicase activities in the same polypeptide chain. Subunits of the heptameric crystal structure of gp4B (PDB entry 1q57 (ref.49) were aligned with the hexameric helicase fragment (PDB ID code: 1e0k (ref.30) and primase fragment (PDB entry 1 nui (ref.50) of gp4. Schematic representation of gp4 constructs (bottom). The boundaries for the helicase and primase domains of gp4 are depicted51. The three constructs containing the C-terminal helicase domain of gp4 are denoted as gp4A, B and D. Residue numbers are as indicated. The figure was created using PyMOL (http://www.pymol.org). (b) Effect of PEG on oligonucleotide synthesis by primase fragment. The standard reaction contained the oligonucleotide 5′-GGGTCA10-3′ containing the primase recognition sequence, 200 μM [α-32P]-CTP and ATP, and increasing amounts of 1 kDa PEG (0, 1.25, 2.5, 5 and 10%) in a buffer containing 40 mM Tris-HCl (pH 7.5), 10 mM MnCl2, 10 mM DTT and 50 mM potassium glutamate. The quenched samples were loaded onto 25% polyacrylamide sequencing gel containing 3 M urea and visualized using autoradiography. (c) Effect of PEG on the DNA unwinding activity of gp4B. The DNA fork depicted (right) was prepared by partially annealing a 5′-32P labelled 45-mer oligonucleotide to a 65-mer oligonucleotide. DNA unwinding activity was performed in a standard reaction containing 40 mM Tris-HCl (pH 7.5), 50 mM potassium glutamate, increasing amounts of PEG 1 kDa (0, 0.25, 0.5, 1, 2, 4 and 8%) and 400 nM of gp4B. The gel shows the separation of unwound ssDNA (bottom) from the dsDNA substrate in a 10% non-denaturing gel. (d) Effect of highly crowding conditions (8% PEG) on the DNA-dependent dTTPase activity of gp4B. The dTTPase activity was measured in the presence of 5 mM dTTP and 8% PEG and with various concentrations of gp4B (0–200 nM). Difference in the dTTPase activity in the presence and absence of high concentration of PEG is denoted as residual. Figure 3: The effect of macromolecular crowding on gp4 activity. ( a ) Front (top panel) and side view (middle panel)of a gp4 model. Gp4 has both primase and helicase activities in the same polypeptide chain. Subunits of the heptameric crystal structure of gp4B (PDB entry 1q57 (ref. 49 ) were aligned with the hexameric helicase fragment (PDB ID code: 1e0k (ref. 30 ) and primase fragment (PDB entry 1 nui (ref. 50 ) of gp4. Schematic representation of gp4 constructs (bottom). The boundaries for the helicase and primase domains of gp4 are depicted [51] . The three constructs containing the C-terminal helicase domain of gp4 are denoted as gp4A, B and D. Residue numbers are as indicated. The figure was created using PyMOL ( http://www.pymol.org ). ( b ) Effect of PEG on oligonucleotide synthesis by primase fragment. The standard reaction contained the oligonucleotide 5′-GGGTCA 10 -3′ containing the primase recognition sequence, 200 μM [α- 32 P]-CTP and ATP, and increasing amounts of 1 kDa PEG (0, 1.25, 2.5, 5 and 10%) in a buffer containing 40 mM Tris-HCl (pH 7.5), 10 mM MnCl 2 , 10 mM DTT and 50 mM potassium glutamate. The quenched samples were loaded onto 25% polyacrylamide sequencing gel containing 3 M urea and visualized using autoradiography. ( c ) Effect of PEG on the DNA unwinding activity of gp4B. The DNA fork depicted (right) was prepared by partially annealing a 5′- 32 P labelled 45-mer oligonucleotide to a 65-mer oligonucleotide. DNA unwinding activity was performed in a standard reaction containing 40 mM Tris-HCl (pH 7.5), 50 mM potassium glutamate, increasing amounts of PEG 1 kDa (0, 0.25, 0.5, 1, 2, 4 and 8%) and 400 nM of gp4B. The gel shows the separation of unwound ssDNA (bottom) from the dsDNA substrate in a 10% non-denaturing gel. ( d ) Effect of highly crowding conditions (8% PEG) on the DNA-dependent dTTPase activity of gp4B. The dTTPase activity was measured in the presence of 5 mM dTTP and 8% PEG and with various concentrations of gp4B (0–200 nM). Difference in the dTTPase activity in the presence and absence of high concentration of PEG is denoted as residual. Full size image The effect of macromolecular crowding on primase and helicase activities was examined ( Fig. 3b ). On a DNA template containing the primase recognition site 5′-GGGTC-3′, the primase fragment catalyses the synthesis of the di-, tri- and tetraribonucleotides pppAC, pppACC and pppACCC [28] . We examined the synthesis of oligoribonucleotides in the presence of PEG. The reaction conditions involve incubating the primase fragment (gp4 residues 1–271, 30 kDa) with an oligonucleotide containing a primase recognition sequence, [α- 32 P] CTP and ATP, and increasing amounts of PEG (0–10%). The radioactively labelled oligoribonucleotide are separated on a denaturing polyacrylamide gel and the radioactivity measured on an autoradiogram. Macromolecular crowding does not affect tetramer synthesis but slightly enhances trinucleotide formation ( Fig. 3b ). In the unwinding assay, a radiolabeled DNA strand partially annealed to a complementary strand creates a fork structure (see cartoon in Fig. 3c ). Unwinding of the DNA releases the radiolabeled strand that has a mobility in 10% TBE gels greater than that of the fork structure. In the experiment, ( Fig. 3c ) the DNA was incubated with 400 nM gp4B, dTTP and increasing amounts of PEG 1 kDa (0–8%). Increasing amounts of PEG results in enhancement of unwinding activity as observed by the radiolabeled DNA strand that migrates more rapidly than the fork substrate. Concentrations of PEG >4% result in protein precipitation ( Fig. 3c , lane 8). The DNA-dependent dTTP hydrolysis activity of gp4B in 8% PEG was examined ( Fig. 3d ). At this high concentration of PEG the dTTP hydrolysis activity of gp4B is enhanced up to 70 nM of the enzyme. The dotted line represents the theoretical activity taking the excluded volume effect of PEG into account. The activity in the presence of PEG is higher than that predicted, suggesting that excluded volume is not the only factor contributing to the increased activity. Increasing amounts of PEG enhances not only the DNA-dependent dTTPase activity but also the DNA-independent dTTPase ( Supplementary Fig. S1b ), presumably owing to an enhancement of oligomerization of gp4B. Macromolecular crowding enhances the concerted activity of gp4 and gp5/trx Leading- and lagging-strand synthesis involves interactions between gp5/trx and the helicase and primase. On the leading strand, the helicase activity unwinds the DNA ahead of gp5/trx to which it is tightly bound. The effect of PEG on leading-strand synthesis was measured using circular M13 DNA containing a replication fork ( Fig. 4a , top). Gp5/trx and gp4B (helicase but no primase activity) carry out strand-displacement synthesis ( Fig. 4a ). The addition of increasing amounts of PEG increases the rate of DNA synthesis with a three-fold increase occurring at 4% PEG. 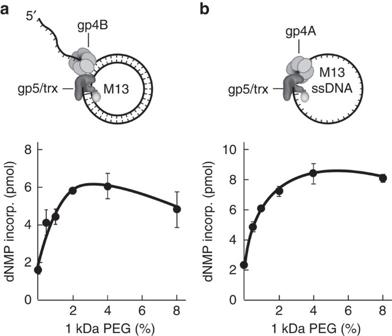Figure 4: The effect of macromolecular crowding on gp5/trx and gp4 interactions. The three proteins move the replication fork at a rate of approximately 150 nt per second at 25°. The bifunctional gene 4 helicase-primase (gp4) assembles on the lagging strand as a hexamer, where it forms a complex with gp5/trx and unwinds the DNA duplex. (a) Effect of PEG on strand-displacement DNA synthesis mediated by gp5/trx and gene 4 helicase (gp4B). Using M13 dsDNA with a 5′-ssDNA tail (top), the efficiency of strand-displacement DNA synthesis in the presence of PEG was determined. The standard reaction contained the dsM13 template (10 nM), 0.3 mM dATP, dGTP, dCTP and [α-32P] dTTP (0.1 μCi), 10 nM gp5/trx, 200 nM monomeric concentrations of gp4B and increasing amounts of PEG 1 kDa (0–8%). After incubation for 30 min at 37 °C and the amount of DNA synthesis was determined by the amount of [α-32P] dTTP incorporated into DNA. (b) Primase-dependent DNA synthesis. The reaction was similar toaexcept that gp4A replaced gp4B and 10 nM M13 ssDNA replaced the dsM13 DNA. The reaction buffer also contained ATP and CTP (100 μM each). The amounts of primase-dependent DNA synthesis was determined by measuring the incorporation of [32P] dTMP into DNA. The error bars were derived from three independent experiments. Figure 4: The effect of macromolecular crowding on gp5/trx and gp4 interactions. The three proteins move the replication fork at a rate of approximately 150 nt per second at 25°. The bifunctional gene 4 helicase-primase (gp4) assembles on the lagging strand as a hexamer, where it forms a complex with gp5/trx and unwinds the DNA duplex. ( a ) Effect of PEG on strand-displacement DNA synthesis mediated by gp5/trx and gene 4 helicase (gp4B). Using M13 dsDNA with a 5′-ssDNA tail (top), the efficiency of strand-displacement DNA synthesis in the presence of PEG was determined. The standard reaction contained the dsM13 template (10 nM), 0.3 mM dATP, dGTP, dCTP and [α- 32 P] dTTP (0.1 μCi), 10 nM gp5/trx, 200 nM monomeric concentrations of gp4B and increasing amounts of PEG 1 kDa (0–8%). After incubation for 30 min at 37 °C and the amount of DNA synthesis was determined by the amount of [α- 32 P] dTTP incorporated into DNA. ( b ) Primase-dependent DNA synthesis. The reaction was similar to a except that gp4A replaced gp4B and 10 nM M13 ssDNA replaced the dsM13 DNA. The reaction buffer also contained ATP and CTP (100 μM each). The amounts of primase-dependent DNA synthesis was determined by measuring the incorporation of [ 32 P] dTMP into DNA. The error bars were derived from three independent experiments. Full size image Lagging-strand synthesis requires gp4A, the full length gp4, for the synthesis of olioribonucleotides to initiate the synthesis of Okazaki fragments [28] . To examine the synthesis of primers and their transfer to gp5/trx we have used M13 ssDNA for the primase to synthesize oligoribonucleotides and for gp5/trx to extend the primers ( Fig. 4b , top). In this assay, the full-length gp4 (gp4A) was used. To initiate DNA synthesis the primase must first synthesize tetraribonucleotides on the DNA and then transfer them to gp5/trx. ATP and CTP are provided in addition to the four dNTPs as the primers synthesized are pppACCC, pppACAC and pppACCA. As shown in Fig. 4b primase-dependent DNA synthesis increases up to four-fold upon the addition of PEG 1 kDa. However, oligoribonucleotide synthesis is not affected ( Fig. 3b ). The decrease of both strand-displacement DNA synthesis and primase-dependent DNA synthesis at PEG concentration above 4% is due to precipitation of the proteins ( Supplementary Fig. S2 ). Macromolecular crowding makes gp5/trx–gp4 complex more compact During the leading-strand synthesis, gp5/trx and gp4 form a stable complex that increases processivity [16] . Two interactions of gp5/trx and gp4 are responsible for this increase in processivity. A tight interaction of the two proteins results in a processivity of approximately 5,000 nt. The processivity is limited to 5,000 nt by the occasional dissociation of gp5/trx. A second interaction of the C-terminal tail of gp4 with a basic patch on gp5 captures gp5/trx in the event in which it dissociates and allows it to return to the primer, increasing the processivity to >17,000 nt. We have used SAXS to examine the structure of this later complex and to determine the effect of macromolecular crowding on the complex. Gp4D (residues 241–566, 36 kDa) is the minimal fragment of the helicase that forms hexameric rings ( Fig. 3a , grey). Gp4D contains the helicase domain and the linker connecting the helicase and primase domains. Although gp4D has less helicase activity than that of gp4A or gp4B it forms stable hexamers in the presence of ssDNA and dTTP and it binds gp5/trx at the replication fork to form a stable complex [29] . All of the features of gp4D and its available hexameric crystal structure [30] facilitate solution structural experiments using SAXS. To assure the stability of the hexamer of gp4D we have used a 15 nt oligonucleotide to which gp4D binds tightly in the presence of the non-hydrolyzable analogue β,γ methylene dTTP (ref. 31 ). It is crucial to ascertain that the complex between gp5/trx and gp4D can be identified before the addition of PEG. Therefore, we carried out SAXS analysis on samples containing a constant amount of gp4D but increasing amounts of gp5/trx. This procedure enables the detection of weakly interacting high molecular weight protein complexes. We recently applied this method to translation initiation complexes [32] . This method also provides information on the stoichiometry of proteins within the complex. As shown in the scheme presented in Fig. 5a , mixing of two interacting proteins will result in an increase at the R g values. The amount of one protein needed to obtain saturation of the R g value provides information on the tendency of the species to form a complex. Thus, strong complexes are characterized by a sharp rise of the R g value until saturation with only small amount of protein that is titrated over the other, and vice versa. If the proteins do not form a complex the R g value represents an intermediate value of the two. 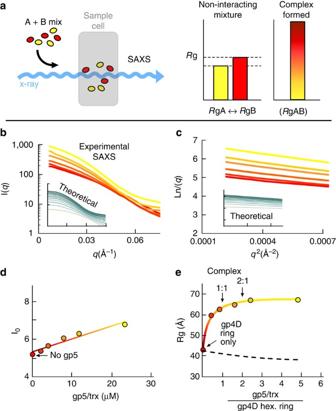Figure 5: SAXS reconstitution assay of the gp5/trx/gp4D complex. (a) Schematic view of the experimental design. Samples containing proteins A and B are premixed in various ratios and placed in the sample cell.Rgvalues were extracted from the SAXS data. IncreasedRgvalues indicate that a higher-order species is formed. IntermediateRgvalue from the individual proteins in the mixture is indicative of non-interacting species. (b,c) Small-angle X-ray scattering (SAXS) curves of gp4D (5 μM) premixed with increasing amounts of gp5/trx (0, 2, 4, 8, 12 and 24 μM). Raw SAXS data (b) and the corresponding Guinier plots (c) for every sample. Colours indicate a gradual increase in the gp5/trx concentration (red to yellow). (c) TheRgvalues for the complex formed derived from these data and determined using Guinier plots. The insets in bothb,crepresent the theoretical SAXS curves of linearly combined spectra (from the available crystal structures) of the putative complex and the free proteins in solution. The data represent a complex between hexameric gp4D and gp5/trx in a molar ratio of 1:2, respectively. The theoretical SAXS curves of gp4D bound to gp5trx in a molar ratio of 1:1, 1:2, 1:3 and 1:4, respectively, are presented inSupplementary Fig. S4. (d) Scattering intensities (I0) shown as a function of concentration of gp5/trx. Data present scattering at zero angle of gp4D (5 μM) and increasing amounts of gp5/trx (0–24 μM), corresponding to the amount of electron scatterers at any sample. (e) SAXS results plotting the radius of gyration (Rg) against gp5/trx and gp4D ratios. Experimental SAXS data were collected for gp4D (5 μM) and increasing amounts of gp5/trx (0–24 μM) in a buffer containing 20 mM Tris-HCl (pH 7.5), 50 mM potassium glutamate and 2 mM DTT. Gp4D was premixed with 6.6 μM 15-mer ssDNA and 0.5 mM β, γ methylene dTTP to form hexameric molecules.Rgserves as an indicator for the formation of higher-order protein complexes. The dashed line represents a theoretical curve ofRgvalues that would be obtained if the components did not interact. Figure 5: SAXS reconstitution assay of the gp5/trx/gp4D complex. ( a ) Schematic view of the experimental design. Samples containing proteins A and B are premixed in various ratios and placed in the sample cell. R g values were extracted from the SAXS data. Increased R g values indicate that a higher-order species is formed. Intermediate R g value from the individual proteins in the mixture is indicative of non-interacting species. ( b , c ) Small-angle X-ray scattering (SAXS) curves of gp4D (5 μM) premixed with increasing amounts of gp5/trx (0, 2, 4, 8, 12 and 24 μM). Raw SAXS data ( b ) and the corresponding Guinier plots ( c ) for every sample. Colours indicate a gradual increase in the gp5/trx concentration (red to yellow). ( c ) The R g values for the complex formed derived from these data and determined using Guinier plots. The insets in both b , c represent the theoretical SAXS curves of linearly combined spectra (from the available crystal structures) of the putative complex and the free proteins in solution. The data represent a complex between hexameric gp4D and gp5/trx in a molar ratio of 1:2, respectively. The theoretical SAXS curves of gp4D bound to gp5trx in a molar ratio of 1:1, 1:2, 1:3 and 1:4, respectively, are presented in Supplementary Fig. S4 . ( d ) Scattering intensities ( I 0 ) shown as a function of concentration of gp5/trx. Data present scattering at zero angle of gp4D (5 μM) and increasing amounts of gp5/trx (0–24 μM), corresponding to the amount of electron scatterers at any sample. ( e ) SAXS results plotting the radius of gyration ( R g ) against gp5/trx and gp4D ratios. Experimental SAXS data were collected for gp4D (5 μM) and increasing amounts of gp5/trx (0–24 μM) in a buffer containing 20 mM Tris-HCl (pH 7.5), 50 mM potassium glutamate and 2 mM DTT. Gp4D was premixed with 6.6 μM 15-mer ssDNA and 0.5 mM β, γ methylene dTTP to form hexameric molecules. R g serves as an indicator for the formation of higher-order protein complexes. The dashed line represents a theoretical curve of R g values that would be obtained if the components did not interact. Full size image The R g values, corresponding to the size of the measured particles, were derived from the Guinier plots ( Fig. 5c ) that represent the linear small-angle part of the X-ray scattering data ( Fig. 5b ). A typical binding curve is observed upon plotting of R g against the ratio between gp5/trx and gp4D providing information on complex formation ( Fig. 5e ). The R g values are saturated above the ratio of 2:1 for gp5/trx to gp4D hexameric ring, suggesting at least 2 gp5/trx per hexamer ( Fig. 5e ). I 0 is proportional to the molecular mass (number of atomic scatterers). An increase in I 0 owing to the increase in the molecular mass is observed ( Fig. 5d ). There is no evidence of aggregation from Guinier analysis ( Fig. 5c ). We have linearly combined artificial SAXS data to merge the contribution of a theoretical SAXS signal of the complex and the individual proteins ( Supplementary Fig. S4 ). The artificial SAXS data were generated using CRYSOL [33] from the crystal structure of gp5/trx (PDB ID code: 1t8e (ref. 34 ) and gp4D (PDB ID code: 1e0k (ref. 30 ) and a model of the complex. These artificial SAXS spectra serve as a reference for the reconstitution using SAXS to determine how many gp5/trx are bound to one hexameric gp4D. The settings of a theoretical complex by which two polymerases are bound to one helicase hexameric ring fit the data. The effect of PEG on the structure of gp4D and gp5/trx in solution was examined by SAXS. No change in the R g of gp4D or gp5/trx is observed upon titration PEG to the sample ( Supplementary Fig. S3 ) indicating that there is no conformational transition of the individual proteins by PEG. R g of gp5/trx (without primer-template DNA or nucleotides) mixed with gp4D at the ratio of 1:1 is equal to 63 Å ( Fig. 5e ). This R g value fits well with the dimension obtained from a structural model of the complex constructed by the crystal structures of gp5/trx and gp4D [29] . 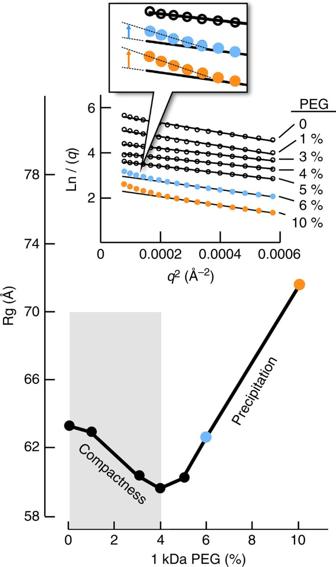Figure 6: The effect of PEG 1 kDa on theRgof gp4D bound to gp5/trx. The sample contained 4.5 μM gp4D (hexamer) premixed with 6.6 μM 15-mer ssDNA, 0.5 mM β, γ methylene dTTP and 5 μM gp5/trx. The reaction buffer contained 20 mM Tris-HCl (pH 7.5), 50 mM potassium glutamate, 2 mM DTT and increasing amounts of PEG 1 k (0–10%). TheRgvalues for the samples were derived from the SAXS data and determined using Guinier plots. SAXS Guinier plots at high PEG concentrations are presented in the inset. Figure 6 shows the R g values of the complex formed with a mixture of gp4D hexamer and gp5/trx at a ratio of 1:1 and increasing amounts of PEG (0–10%). Up to 4% PEG, there is a gradual decrease in the R g indicating compactness of the volume of the gp5/trx–gp4 complex ( Fig. 6 ). The results demonstrate conformational changes in the complex as a result of macromolecular crowding. Figure 6: The effect of PEG 1 kDa on the R g of gp4D bound to gp5/trx. The sample contained 4.5 μM gp4D (hexamer) premixed with 6.6 μM 15-mer ssDNA, 0.5 mM β, γ methylene dTTP and 5 μM gp5/trx. The reaction buffer contained 20 mM Tris-HCl (pH 7.5), 50 mM potassium glutamate, 2 mM DTT and increasing amounts of PEG 1 k (0–10%). The R g values for the samples were derived from the SAXS data and determined using Guinier plots. SAXS Guinier plots at high PEG concentrations are presented in the inset. Full size image We have examined the effect of macromolecular crowding on several of the reactions that occur at the replication fork. Addition of PEG cancels the inhibitory effect of salt on the activity of DNA polymerase (gp5/trx). This effect probably results from an increase in the surface of interaction with DNA, an interaction crucial for increasing processivity [27] . Traditionally, reconstitution of the gp5/trx complex has used a molar excess of trx although the reported Kd for trx binding to gp5 is 5 nM (ref. 35 ). It is now evident that the requirement for an excess of trx is due to macromolecular crowding at higher protein concentration. The use of an inert crowding agent such as PEG or bovine serum albumin can eliminate the need for excessive concentrations of trx. The active site in the helicase where hydrolysis of dTTP occurs is formed at the interface of two subunits (Rec A-like domains). Consequently, the helicase hexamer has a total of six active site clefts where nucleotides bind. PEG increases the efficiency of hydrolysis of dTTP and unwinding activity of the helicase. Does the increase in dTTPase activity result from an apparent increase of gp4 concentration? To answer this question we used 8% PEG to provide a high crowing environment and examined the DNA independent and the DNA-dependent dTTPase activity of gp4B. The apparent concentration of gp4 increased from 70 to 76 nM as the PEG concentration increased from 4 to 8% resulting in a decrease in volume of 8% (see Fig. 1b ). In this new apparent concentration of gp4, the DNA-dependent dTTPase activity increased two-fold. Therefore, the increase in the DNA-dependent dTTPase activity is not governed only by the increase in the apparent concentration of gp4B but also by an increase in hexamer formation. Macromolecular crowding affects the two activities of gp4 differently although both activities reside in the same polypeptide chain. PEG does not increase tetraribonucleotide synthesis by primase fragment while increasing helicase activity. Interestingly, primer synthesis of primase fragment is not affected by PEG, whereas utilization of ATP/CTP is increased (trimer formation) presumably owing to an increase in the affinity of the primase to ATP/CTP. The weak binding of the primase fragment lacking the helicase domain to a DNA template has been observed previously using surface plasmon resonance [36] . The molecular basis for sequence recognition has not yet been elucidated. However, the negligible effect of PEG may indicate transient association and dissociation of the primase to its DNA template, a process affected by diffusion. In the context of the full-length gp4, the priming activity is no longer bimolecular, and, therefore the influence of crowding is expected to be negligible. The effect of PEG on strand-displacement and primase-dependent DNA synthesis along with SAXS analysis of the structures suggest that addition of PEG promotes the association of gp4 to gp5 to form a stable replisome. Protein folding and protein–protein interactions are driven by the same forces. These processes are governed by hydrophobic interactions (polymerization mode), salt-dependent polar (electrostatic mode) and hydrogen–bond interactions. To adapt to environmental stress, cells have evolved an array of effective countermeasures. Osmotic stress is counterbalanced by ‘osmolytes’, small, charged or polar solutes that balance the stress. One direct effect of osmotic stress is that protein side chains are affected by water depletion [37] . Charged residues must search for other interactions when water is absent leading to interactions with other charged residues. We have found, using NMR, that the relaxation of protein residues is affected by macromolecular crowding presumably due to water depletion (Akabayov et al ., manuscript submitted). The loss of conformational entropy in a protein during folding or complex formation is an outcome of the release of water molecules to minimize exposure of hydrophobic patches to solvent [38] . Therefore, water has a central role in protein assembly and thermodynamics is the driving forces involving the motion of water molecules. Release of water molecule by PEG increases the entropy that compensates for the decrease in the entropy upon complex formation. The depletion of water from both DNA polymerase and DNA helicase would presumably increase the contact interaction to DNA and alter the conformation of the protein to enhance its movement on DNA. Another challenge is to characterize the structure of weakly binding protein counterparts. Traditionally, attention has been directed toward the structure of stable complexes of macromolecules. Most biophysical characterizations are dependent on the acquisition of a stable species, a requirement not easily met with weakly interacting macromolecules. Interest in the structure of weakly interacting components in complexes has risen significantly over the years, particularly with regard to the high molecular weight transient complexes involving DNA replication. Weak interactions between T7 DNA polymerase and gp4 are not short lived [39] . We assume that complex formation between DNA polymerase and gp4 remain stable (although governed by weak interactions) to enable copying the entire genome. We have shown how SAXS can be used to probe high molecular weight complexes such as a gp5/trx–gp4. The number of DNA polymerases in a functional replisome is not known. SAXS can provide an estimate of the stoichiometry of gp5/trx on a hexamer of gp4D within a reconstituted complex. We have used SAXS to determine the number of gp5/trx molecules bound to a hexamer of gp4 when neither protein is in a replication mode. Such a complex represents that formed the replication fork and involves the C-terminal tail of gp4 and a basic patch on gp5/trx. It is this complex that provides a backup gp5/trx in the event that gp5/trx dissociates into solution, an exchange that assures processivity. Our data supported by linear combination analysis of theoretical SAXS spectra show that there are two DNA polymerases per hexamer of gp4. The leading- and lagging-strand gp5/trx are bound via different interactions and would thus add two more gp5/trx to the replisome. Using this SAXS-based assay we have determined the best conditions for subsequent experiment with PEG. We have used a similar approach to characterize the interactions between the C-terminal domain of eIF5 and eIF1 (ref. 32 ). This approach is not necessarily limited to SAXS. We have identified interactions of Mn-dNTP to the active site of T7 DNA polymerase using X-ray absorption near edge spectroscopy utilizing the same principle [40] . In the later experiment, we were able to distinguish between signal originating from Mn 2+ that is free in solution and Mn 2+ bound to the active site of gp5. These methods together with biochemical and other biophysical methods provide an opportunity to investigate the structure of high molecular weight complexes that cannot be crystallized owing to weak binding interactions or have size limitations for NMR. Although there is considerable information on the effect of macromolecular crowding on bimolecular reaction there is little information on its effect on the structure of the molecules involved. FlgM, an unstructured protein folds to adopt a structure in a macromolecular-crowded environment [41] . Likewise, the two unrelated proteins: VlsE and α/β flavodoxin increase their structural content by folding of the unstructured regions [7] . We have shown that the complex between gp5/trx and gp4D adopts a compact conformation in an environment with macromolecular crowding. We suggest that crystal structure or NMR solution structures may not represent precisely the in vivo structure if no consideration of the macromolecular crowding effect is taken into account. Protein expression and purification Chemicals were from Sigma. ATP and CTP were from Roche Molecular Biochemicals. dNTPs were from USB Corp. Pre-made gels (10–20% linear gradients) were from BioRad (Hercules, CA). T7 gp5, gp4, E. coli trx were overproduced and purified as described [26] , [42] . M13 ssDNA was prepared as described previously [43] . [γ– 32 P] dATP (800 Ci mmol −1 ), [α– 32 P] CTP and dTTP (800 Ci mmol −1 ) were from Perkin Elmer. DNA unwinding assay The unwinding activity of gp4 was measured using a mini replication fork consisting of 5′ 32 P-labelled 45-mer oligonucleotide (5′-ATGACTCTATGCACATTGACATGCTTCAGATTCGTATTGTACACT-3′) partially annealed to a 65-mer oligonucleiotide (5′-T 20 AGTCGTAATCCGACCTCGAGGCATTGTCAATGTGCATAGAGTCAT-3′). Reactions contain 400 nM monomeric gp4B, 100 nM DNA, 40 mM Tris-HCl (pH 7.5), 10 mM MgCl 2 , 0.1 mM DTT, 50 mM potassium glutamate, 1 mM dTTP and the indicated concentrations of PEG 1 kDa. The reaction was incubated for 5 min at 37 °C and terminated by adding 5 × stop buffer to a final concentration of 0.4% SDS, 40 mM EDTA, 8% glycerol and 0.1% bromophenol blue. Samples were loaded onto 10% non-denaturing polyacrylamide gel. The amount of radiolabeled single stranded 45-mer formed was measured using a Fuji BAS Bioimaging analyser. dTTPase activity The dTTPase activity of gp4 was determined in a reaction containing 0–200 nM gp4B, 1 nM M13 ssDNA, 5 mM dTTP, 0.1 mCi of [α– 32 P] dTTP, 40 mM Tris-HCl (pH 7.5), 10 mM MgCl 2 , 50 mM potassium glutamate, 0.1 mM DTT and 8% PEG 1 kDa. After 10 min at 37 °C, the reaction was halted using 40 mM EDTA and 0.4 μl was spotted onto polyethyleneimine TLC plate (EMD). Reaction products were separated using 0.5 M formate and 0.5 M LiCl. The plate was dried, subjected to autoradiography and the products measured. Oligoribonucleotide synthesis Synthesis of oligoribonucleotides by primase was measured as described [44] in reactions containing 5 μM T7 primase fragment. Reactions (10 μl) contained 5 μM DNA templates (5′-GGGTCA 10 -3′), 200 μM ATP, 200 μM [α- 32 P]-CTP, primase fragment, 40 mM Tris-HCl pH 7.5, 10 mM MnCl 2 , 10 mM DTT, 50 mM potassium glutamate and 1 kDa PEG (0, 1.25, 2.5, 5 and 10%). After incubation at room temperature for 10 min, the reaction was terminated by adding an equal volume of sequencing buffer containing 98% formamide, 0.1% bromophenol blue and 20 mM EDTA. The samples were loaded onto 25% polyacrylamide sequencing gel containing 3 M urea and visualized using autoradiography. DNA polymerase assay Polymerase activity was measured in a reaction containing 20 nM M13 ssDNA annealed to a 24-mer primer, 40 mM Tris-HCl (pH 7.5), 10 mM MgCl 2 , 10 mM DTT, 50 mM potassium glutamate, 0.25 mM dTTP, dGTP, dCTP and [α– 32 P] dATP (5 cpm pmol −1 ). Gp5 (or gp5/trx) and PEG 1 kDa were added at the indicated amount. The reaction was incubated at 37 °C for 10 min and terminated by the addition of EDTA to 40 mM. Aliquots were spotted on DE-81 filters (Whatman), washed extensively with 0.3 M ammonium formate (pH 8.0) and the radioactivity retained measured. Strand-displacement synthesis DNA templates were prepared by annealing a primer containing 5′ non-complementary ssDNA region (underlined) (5′- T 36 AATTC GTAAT CATGG TCATAGCTGT TTCCT-3′) to M13 DNA. The reaction contained 10 nM template DNA, 0.3 mM dNTPs, 0.1 μCi [α– 32 P] dTTP, 20 nM T7 gp5/trx, 200 nM gp4B and the indicated concentrations of PEG 1 kDa. The reaction was incubated for 30 min at 37 °C and the amount of DNA synthesis determined as in the polymerase assay. Primase-dependent DNA synthesis RNA primers made by gp4A were extended by gp5/trx. The reaction contained 10 nM M13 ssDNA, 0.3 mM dNTPs, 0.1 μCi [α– 32 P] dCTP, 20 nM gp5/trx, 200 nM monomeric gp4A and PEG 1 kDa (0–8%). The reaction was incubated for 30 min at 37 °C and amounts of DNA synthesis were determined as described in the polymerase assay. Small-angle X-ray scattering (SAXS) Measurements were made at the National Synchrotron Light Source (Upton, NY) on beamline X-9. Sample loading, data collection and processing were performed as described [45] . The magnitude of the scattering vector ( q ) is defined as: where 2 θ is the scattering angle. The SAXS data showed a linear behaviour ( see Fig. 5c and Fig. 6 —except samples containing 6 and 10% PEG) in the low q , Guinier region, indicating that the proteins did not aggregate. R g were derived from data in the q R g <1.3 region using the Guinier approximation embedded in PRIMUS 46 : To ensure binding of gp5/trx to gp4D we used samples prepared as followed. Binding of gp5/trx ( A ) to gp4D ( B ) is a single-step reaction of the type A + B ⇄ AB . The dissociation constant is given by Where [ A ] is the concentration of gp5/trx and [ B ] is the concentration of gp4D hexamers and [ AB ] is the concentration of the complex in equilibrium. Expressing the equilibrium concentrations of the separate components in terms of initial concentrations (indicated by a subscript Zero) and the concentration of the complex We obtain If we wish to have x fraction of A 0 in the complex AB : Then the following amount of B is required to have AB complex: B 0 , the concentration of gp4D was kept constant at 5 μM for all samples; K D , the dissociation constant is 90 nM (ref. 39 ). Therefore, to obtain a 1:1 complex, 5.3 μM gp5/trx was mixed with 5 μM gp4D. To examine whether binding of multiple gp5/trx occur per one hexamer of gp4D, gp5/trx with various concentrations (0, 2, 4, 8, 12 and 24 μM) was added. The components were mixed before the SAXS measurement, centrifugated for 1 min to eliminate scattering from precipitated protein and measured. The samples of gp5/trx and gp4D were measured in 20 mM Tris-HCl (pH 7.5), 50 mM potassium glutamate, 2 mM DTT. To simulate the scattering profile and R g for a mixture of gp5/trx and gp4D, we calculated the scattering intensity using the following formula: with q =scattering vector, I 0 is the extrapolated intensity at zero scattering angle, R g , the radius of gyration of the respective particle. The intensity at zero scattering angle was calculated according to where N is the number of particles per unit volume and V the volume of the particle with: The apparent R g of the mixture was then calculated from slope of the curve of ln( I ) versus q 2 according to the Guinier approximation: NMR Spectroscopy We carried out DOSY-NMR experiments using a stimulated spin echo sequence on lysozyme in the presence or the absence of PEG to evaluate the effect of PEG on diffusion coefficients. The decrease in magnetization with increasing gradient strength can be analysed using the following formula: where D is the diffusion coefficient with k B is the Boltzmann constant, T the temperature, η the viscosity, F the dimensionless Perrin factor, r S the hydrodynamic radius of the molecule q=γδg , Δ is the separation of the gradient echo, δ the gradient duration, γ the gyromagnetic ratio of the nucleus and g the strength of the gradient. The duration of the gradient in this experiment was set to 2.5 ms, the separation of the gradient echo to 150 ms. The gradient strength was varied from 15 to 80 G cm −1 . Thirty two points were recorded in the indirect dimension. DMSO was used as an internal reference. Simulation of Brownian motion We used Matlab to perform a simple simulation of Brownian motion in a space of the size of an E. coli cell with and without ribosomes as crowding agents. We calculated 18,000 random positions of non-overlapping spheres with a radius of 11 nm in E. coli. cell space (0.8 × 2 μm 2 ). We used the diffusion coefficient with k B =Boltzmann constant, T =temperature (293 K), η =viscosity inside an E. coli cell with η =3.5 × 10 −3 kg m −1 s −1 (ref. 47 ) and d =radius of the particle, here d =30 Å, to calculate the average displacement squared with k= 2 Dnτ , where D is the diffusion coefficient, n the number of dimensions (3) and τ the time interval (here 0.0001, s). The displacement vector for each time interval was determined by multiplying a random number by the displacement factor using Matlab’s random function for normal distribution of random numbers. If the new position of the molecule overlapped with a ribosome position of if the position was outside the confines of the given space, a new position was calculated in the same manner. For simplicity, the positions of the ribosome molecules were kept fixed. Excluded volume calculation To calculate the excluded volume, we assumed spherical shape of the PEG molecules. The specific volume was calculated using the following equation with r h =hydrodynamic radius, N A =Avogadro constant, MW=molecular weight. To calculate the volume occupied by PEG at different concentrations, the specific volume is multiplied by the density of PEG and the concentration. The values for the hydrodynamic radius of PEG with different sizes was taken from ref. 47 . How to cite this article: Akabayov B. et al . Impact of macromolecular crowding on DNA replication. Nat. Commun. 4:1615 doi: 10.1038/ncomms2620 (2013).